A scalable method for preparing Cu electrocatalysts that convert CO2into C2+products Development of efficient catalysts for selective electroreduction of CO 2 to high-value products is essential for the deployment of carbon utilization technologies. Here we present a scalable method for preparing Cu electrocatalysts that favor CO 2 conversion to C 2+ products with faradaic efficiencies up to 72%. Grazing-incidence X-ray diffraction data confirms that anodic halogenation of electropolished Cu foils in aqueous solutions of KCl, KBr, or KI creates surfaces of CuCl, CuBr, or CuI, respectively. Scanning electron microscopy and energy dispersive X-ray spectroscopy studies show that significant changes to the morphology of Cu occur during anodic halogenation and subsequent oxide-formation and reduction, resulting in catalysts with a high density of defect sites but relatively low roughness. This work shows that efficient conversion of CO 2 to C 2+ products requires a Cu catalyst with a high density of defect sites that promote adsorption of carbon intermediates and C–C coupling reactions while minimizing roughness. Combustion of fossil fuels is the leading cause of global warming due to the accumulation of CO 2 in the atmosphere [1] , [2] . The electrochemical CO 2 reduction reaction (CO 2 RR), driven by renewable energy, is a promising strategy to reduce CO 2 accumulation. By converting CO 2 into products of higher value, a closed-loop carbon economy begins to emerge [3] , [4] , [5] , [6] , [7] . To make CO 2 RR economically viable, efficient electrocatalysts with high selectivity for targeted products at scale are needed. Among the metals studied, copper is the only metal known for its intrinsic ability to convert CO 2 into hydrocarbons and alcohols via electrochemical CO 2 RR [3] , [8] . Recent progress at improving the performance of Cu-based electrocatalysts for CO 2 RR has been demonstrated with porous Cu foams [9] , Cu nanoparticle ensembles [10] , oxide-derived Cu [11] , plasma-treated Cu [12] , [13] , Cu nanocubes [13] , [14] , [15] , Cu nanowires [16] , [17] , [18] , wet-oxidation processed CuCl-derived Cu [19] , and single-crystal Cu [20] , [21] . Despite this progress, further advances are needed for producing electrocatalysts at scale that efficiently convert CO 2 into multi-carbon products. As such, the design of catalysts that selectively produce C 2+ products via electrochemical CO 2 RR should focus on minimizing two competing reaction pathways: (1) the hydrogen evolution reaction (HER) and (2) C 1 product formation (e.g., CH 4 , HCOOH). Both pathways reduce the faradaic efficiency (FE) of C 2+ products by consuming electrons and protons. Moreover, C 1 production reduces the amount of adsorbed carbon intermediates available for surface C–C coupling reactions. To minimize HER, the first step of electrochemical CO 2 RR must be enhanced. This first step involves a one electron, one proton reduction of CO 2 to form adsorbed COOH (*COOH) and is a reaction that is affected by the concentration ratio of dissolved CO 2 to protons ([CO 2 ]/[H + ]) near the electrode surface. The relative concentration of dissolved CO 2 and protons near the electrode surface under conditions used for the electrochemical CO 2 RR has been simulated by Gupta et al. and found to be significantly different from bulk concentrations [22] . In addition, Raciti et al. showed that high current densities observed at highly roughened electrocatalysts cause the pH to increase rapidly [17] . Despite the low concentration of protons at high pH, the efficiency of electrochemical CO 2 RR is reduced by the limited availability of dissolved CO 2 on a rough electrode surface. Therefore, to favor electrochemical CO 2 RR over HER, a catalyst with minimal roughness should be used to mitigate a rise in local pH. To minimize C 1 product formation, insights gained from simulations of electrochemical CO 2 RR should guide catalyst design [23] , [24] , [25] , [26] , [27] . These simulations provide an energy landscape that relates the energetics of competing reactions on Cu. For example, the onset potential to form adsorbed CO (*CO) is predicted to be lowest on Cu (211) among the Cu facets simulated: (111), (100), and (211) [25] . Sandberg et al. showed that once *CO forms on a Cu surface, the barrier to forming the C–C coupling product, *OCCO, is lowest on Cu (100) relative to (111) and (211). In addition, the barrier for CO dimerization decreases with increasing *CO coverage [27] . Moreover, C 2 product formation follows second-order kinetics with a rate proportional to the concentration of reactive C 1 intermediates such as *CO. Here, the rate determining step is dimerization of *CO to form C 2 products [28] , [29] , [30] . Other unsaturated C 1 intermediates derived by reduction of *CO (i.e., *CHO, *COH, *CH 2 , and *CHOH) react with *CO to yield C 2+ products [23] , [24] , [26] , [31] , [32] . Thus, high surface coverage of reactive C 1 intermediates is essential and only obtained by a high density of surface defects. Defect sites such as grain boundaries, step sites, and vacancies that result in under-coordinated atoms on the surface of Cu are known to promote C–C coupling [33] , [34] . In addition, Cu + and subsurface oxygen are proposed to promote the adsorption of CO 2 and C–C coupling [12] , [35] , [36] , [37] , [38] , although the stability of subsurface oxygen remains controversial [34] , [35] , [39] , [40] . To maximize the amount of Cu (100) surface, Chen et al. reported cubic microstructures of Cu formed when a Cu foil was cycled between oxidizing and reducing potentials in 0.1 M KCl [41] . Other researchers employed a similar method to prepare Cu catalysts with cubic microstructure and studied product selectivity as a function of plasma-treatment [13] , other halide ions [42] , or stability of residual oxides (indicated by 18 O labeling) [34] . In all cases, the catalysts were more selective for ethylene than methane. However, the FE for C 2 H 4 reported in these studies ranged between 15 and 45%. This difference is likely due to the chemical complexity of the electrochemical cycling method employed. In our hands, the electrochemical cycling method used in previous studies produces only cubic microstructures at oxidizing potentials (Supplementary Fig. 1 ). Advances made in the previous studies inspired us to study each parameter influencing catalyst performance separately (i.e., chemical species present and their reactivity/solubility, applied potential, pH, and roughness) in order to develop a novel electrochemical method that utilizes these parameters to produce a Cu electrocatalyst selective for C 2+ products. In this study, electrocatalysts with a balance of high density of defect sites (i.e., under-coordinated Cu) and low roughness are shown to efficiently convert CO 2 to C 2 and C 3 products (FE C2+ of 72%) via electrochemical CO 2 RR. The electrochemical method used to produce these electrocatalysts consists of three steps: (i) anodic halogenation of Cu foils, (ii) subsequent oxide formation in a KHCO 3 electrolyte, and (iii) electroreduction (Fig. 1 ). Here, chlorinated Cu, brominated Cu, or iodinated Cu were prepared by applying an oxidative potential to Cu foils immersed in 0.1 M KCl, KBr, or KI, respectively, and are henceforth denoted as Cu_KCl, Cu_KBr, and Cu_KI to reflect the different electrolytes used for anodic halogenation. Grazing-Incidence X-ray diffraction (GI-XRD) confirms the presence of Cu(I) halide on the surface of the halogenated Cu foils. Analysis of the morphological and chemical changes by SEM and EDS elucidated the processes by which subsequent surface reconstruction occurs. EDS also provides evidence that subsurface oxygen at the defect sites of Cu_KCl, Cu_KBr, and Cu_KI are produced via oxidation of Cu by high local pH of the electrolyte. The performance of these electrocatalysts provides strong evidence that both a high density of defect sites and low roughness are critical to promoting the formation of C 2+ products via electrochemical CO 2 RR by minimizing competing HER and C 1 production. Fig. 1: Schematics showing morphology of Cu catalysts. a The method used to prepare Cu catalysts for electrochemical CO 2 RR: anodic halogenation in KX solutions where X = halogen, oxide formation in basic KHCO 3 , and electroreduction in neutral KHCO 3 by LSV. EP-Cu corresponds to electropolished Cu foils, LSV corresponds to linear sweep voltammetry. b Two-dimensional visualization of under-coordinated Cu atoms and surface roughness with the corresponding outcomes when used for the electrochemical CO 2 RR. This schematic is simplified but face-centered cubic Cu has a coordination number of 12. Full size image Preparation of electrocatalysts Halogenated Cu foils were prepared by applying an oxidative potential to electropolished Cu foils immersed in an electrolyte containing halide ions. A three-electrode configuration was used: Cu-foil working electrode, Pt gauze counter electrode, and Ag/AgCl reference electrode. The open circuit potential (OCP) of Cu foil immersed in 0.1 M KCl, KBr, or KI aqueous electrolyte was −0.115, −0.134, and −0.315 V vs. Ag/AgCl, respectively (see Supplementary Fig. 2 ). Chronoamperometric potentials of 1.1, 0.18, and −0.2 V vs. Ag/AgCl were applied to a Cu-foil working electrode while immersed in 0.1 M KCl, KBr, or KI, respectively. Note that the working electrode experiences an effective potential ( V eff ) defined as V eff = V app – V oc , where V app is the applied potential and V oc is the measured OCP. For example, an applied potential of −0.2 V vs. Ag/AgCl in 0.1 M KI corresponds to an effective potential of 0.115 V vs. Ag/AgCl, which anodically iodinates the Cu. Current density vs. anodic halogenation time for each electrolyte is shown in Supplementary Fig. 2 . Evaluation of changes in the crystal structure of Cu_KX The crystal structure of Cu foils subjected to anodic halogenation was identified by grazing incident X-ray diffraction (GI-XRD) (Fig. 2 ). Included in this figure is GI-XRD data of control samples: the original electropolished Cu foil (Fig. 2a ) and of electropolished Cu foil after being oxidized in the absence of halide ions (0.05 M K 2 SO 4 aqueous electrolyte, 1.1 V vs. Ag/AgCl, 300 s) (Fig. 2b ). The GI-XRD data of the control sample shows that oxidation in the absence of halide ions produces Cu 2 O on the surface of the Cu foil. In contrast, anodic halogenation of electropolished Cu foils in KCl, KBr, or KI results in the formation of CuCl, CuBr, or CuI, respectively (Fig. 2c–e ). Fig. 2: Crystal structures of halogenated Cu identified by grazing incident X-ray diffraction. GI-XRD patterns of the original electropolished Cu foil ( a ). Cu foils oxidized in 0.05 M K 2 SO 4 at 1.1 V vs. Ag/AgCl for 300 s (control sample) ( b ), or halogenated in KCl ( c ), in KBr ( d ), and in KI ( e ) for 100, 60, and 30 s, respectively. The symbol # indicates peaks corresponding to the underlying Cu-foil substrate. The incidence angle used for GI-XRD was 2°. The inset of each GI-XRD plot is a diagram of the unit cell for Cu, Cu 2 O, CuCl, CuBr, and CuI, from ( a ) to ( e ), respectively. Cu atoms are represented as blue spheres. Source data are provided as a Source data file. Full size image Evaluation of changes in the morphology of Cu_KX The morphology of the Cu foils was expected to change with changes in crystal structure. Therefore, SEM was used to examine samples subjected to anodic halogenation for 50 s (Fig. 3 ). SEM images of samples halogenated for other lengths of time and at different applied potentials are shown in Supplementary Figs. 3 – 7 and SEM images of the control sample are shown in Supplementary Fig. 8 . Cross-sectional images of the samples reveal that a halogenated Cu layer forms on electropolished Cu foils during anodic halogenation in KCl, KBr, or KI for 50 s to a thickness of 1.25, 1.11, and 0.61 μm, respectively (Fig. 3a–c ). Plan-view SEM images of the as-prepared Cu(I) halide are shown in Fig. 3d–f . The formation of a surface layer of Cu(I) halide during anodic halogenation causes a volume expansion that results in surface wrinkling to relieve mechanical stress. This wrinkling is observed in Cu_KCl and Cu_KBr samples but not in the Cu_KI sample, where instead, triangle-based pyramids emerge. Fig. 3: Morphology of halogenated Cu-foil electrodes. SEM images of halogenated Cu foils: a – f as-prepared; g – i after immersion in 0.1 M KHCO 3 for 10 min; j – l after reduction by LSV in the potential range from OCP to −1.8 V in CO 2 -saturated 0.1 M KHCO 3 . a – c Cross-sectional images taken at a tilt angle of 45° to reveal the thickness of halogenated Cu. d – l Plan-view images. Anodic halogenation of Cu was performed for 50 s in 0.1 M KCl at 1.1 V ( a , d , g , j ); in 0.1 M KBr at 0.18 V ( b , e , h , k ); in 0.1 M KI at −0.2 V ( c , f , i , l ). All voltages are reported vs. Ag/AgCl. Scale bars: 2 μm. Full size image The catalysts were subjected to two additional treatments to determine if the morphology of the surface changes further when halogenated Cu foils are immersed in an electrolyte commonly used for CO 2 RR experiments: (1) immersion in air-saturated KHCO 3 , where the pH is basic and (2) electrochemical reduction in CO 2 -saturated KHCO 3 , where the pH is nearly neutral (pH 6.8). These two experiments model the environment that catalysts encounter in preparation for the CO 2 RR but separate the effect of basic pH from that of reducing potentials at near neutral pH. For the first experiment, all Cu_KX samples (where X is a halogen) were immersed in air-saturated 0.1 M KHCO 3 for 10 min. An air-saturated solution of 0.1 M KHCO 3 has a measured pH of 9.0, whose basicity is derived from a shift in equilibrium from bicarbonate ion to its weak acid (H 2 CO 3 ) to produce OH − ions: 
    HCO_3^ -  ( aq)+  H_2O ( aq) ↔H_2CO_3 ( aq) + OH^ -  ( aq)
 (1) When purged with CO 2 (as in the case for the CO 2 RR), the KHCO 3 electrolyte becomes more acidic (pH 6.8) because of the formation of carbonic acid: 
    CO_2 + H_2O ( aq) ↔H_2CO_3 ( aq) ↔H^ +  ( aq)
     +  HCO_3^ -  ( aq) ↔2H^ +  ( aq) + CO_3^2 -  ( aq)
 (2) Based on calculated equilibrium diagrams, Cu 2 O is more stable than CuCl at pH 9 and OCP [43] , [44] . Thus, any morphological changes that may occur when Cu_KX is immersed in KHCO 3 will be caused by an oxide-forming reaction that converts the Cu(I) halide into Cu 2 O: 
    2CuX ( s) +  OH^ -  ( aq) ↔Cu_2O( s) + 2X^ -  ( aq) + H^ +  ( aq)
 (3) In addition, morphological changes should reflect the coordination affinity of copper(I) halides (CuCl < CuBr < CuI) [45] , [46] and their solubility product ( K SP ) in aqueous solution (CuCl > CuBr > CuI) [42] . Consequently, when Cu_KCl is immersed in an air-saturated solution of 0.1 M KHCO 3 (pH 9.0) for 10 min, the relatively unstable CuCl is converted rapidly to Cu 2 O with cubic morphology (Fig. 3g ). The cubic morphology reflects the relative growth kinetics of different facets, where the direction of slowest growth corresponds to the largest facet [47] . Thus, the emergence of cubic morphology during the conversion of CuCl to Cu 2 O suggests that the chloride ions released during this reaction adsorb preferentially on the (100) facet, impeding its growth kinetics. This observation is consistent with simulations that have shown the preferential adsorption of halide ions onto the (100) facet of Cu [48] . When Cu_KBr is subjected to the same treatment, the wrinkled surface of CuBr appears only to shrink slightly from the release of bromide ions into the electrolyte during the oxide-forming reaction [Eq. ( 3 )] (Fig. 3h ). In contrast, when Cu_KI is subjected to the same treatment, the highly stable and insoluble CuI does not undergo any significant morphological change (Fig. 3i ). GI-XRD data further supports the effect of halide ion on the extent to which CuX is converted into Cu 2 O in basic KHCO 3 (see Supplementary Fig. 9 ). These observations are consistent with the trend in stability and solubility of Cu(I) halides and correspond to different rates of oxide formation via [Eq. ( 3 )]. For the second experiment, all Cu foils that had been anodically halogenated and converted to oxide in air-saturated KHCO 3 were reduced by LSV from the measured OCP to −1.8 V vs. Ag/AgCl at a scan rate of 5 mV/s (Supplementary Fig. 10 ). The resulting GI-XRD data (Supplementary Fig. 11 ) is nearly identical to that of the original electropolished Cu, indicating electroreduction by LSV extracts halide ions from the Cu_KX samples. Consequently, reduction of Cu_KCl results in a morphology with smaller but more uniformly sized cubic structures than before (Fig. 3j ) and reduction of Cu_KBr results in further shrinkage and consequential formation of cracks (Fig. 3k ). The reduction of Cu_KI results in a dramatic change to its morphology (Fig. 3i ) and is attributed to the rapid reduction of iodinated Cu: 
    CuI ( s) +  e^ - →Cu ( s) + I^ -  ( aq)
 (4) Recall, Cu_KI does not undergo significant oxide formation in the prior experiment (i.e., immersion in air-saturated KHCO 3 electrolyte). Thus, the electrochemical reduction of Cu_KI causes an abrupt release of iodide ions, leading to the dramatic change in morphology that is observed. In contrast, bromide ions from Cu_KBr are released gradually by the oxide-forming reaction before the sample is subjected to electrochemical reduction. Cu_KCl undergoes relatively rapid oxide formation in KHCO 3 electrolyte so that its morphology has already changed prior to being subjected to electrochemical reduction. Evaluation of changes in the chemical composition of Cu_KX The elemental compositions (Cu, O, and halogen atoms) of the surface of Cu_KX were determined using EDS for the purpose of relating changes in chemical composition to changes in morphology. Raw EDS data are shown in Fig. 4a–d , which can be converted into compositions of molecular species (Fig. 4e–h ) using the chemical species identified by GI-XRD experiments. Details on the conversion of EDS data into chemical species can be found in the Supplementary Information. It is assumed that the halogenated catalysts consist of only three chemical species (i.e., Cu, Cu 2 O, and CuX) because other species such as CuO were not observed in the GI-XRD data (see Supplementary Figs. 9 and 11 ). In the case of electropolished Cu, only two chemical species are assumed to exist: Cu and Cu 2 O. Fig. 4: Energy-dispersive X-ray spectroscopy. a – d Raw data of atomic composition of electropolished Cu foil and halogenated Cu foils as measured by EDS. e – h Compositions of molecular species from converted EDS data. ‘As-prep.’ indicates the as-prepared catalyst by electropolishing or anodic halogenation. ‘Imm.’ indicates the catalyst underwent oxide formation by immersion in air-saturated 0.1 M KHCO 3 electrolyte for 10 min. ‘Reduced’ indicates the catalyst was reduced in CO 2 -saturated 0.1 M KHCO 3 electrolyte by LSV from its corresponding OCP to −1.8 V vs Ag/AgCl at a scan rate of 5 mV/s. Source data are provided as a Source data file. Full size image The initial surface species of Cu_KCl and Cu_KBr are converted into Cu 2 O by the oxide-forming reaction [Eq. ( 3 )] when the samples are immersed in air-saturated 0.1 M KHCO 3 for 10 min (Fig. 4f, g ). For example, EDS data indicates the as-prepared Cu_KCl contains 4.06% of Cu 2 O and 67.3% of CuCl. Similarly, as-prepared Cu_KBr contains 4.13% of Cu 2 O and 66.6% of CuBr. After immersion, rapid oxide formation occurs: Cu_KCl contains 46.2% of Cu 2 O and 12.0% of CuCl while Cu_KBr contains 63.7% of Cu 2 O and 22.4% of CuBr. Unlike Cu_KCl and Cu_KBr samples, Cu_KI showed only slight changes to the composition of the initial surface species due to the high stability of CuI in basic KHCO 3 . The as-prepared sample contained 16.1% of Cu 2 O and 83.9% of CuI whereas the immersed sample contained 21.6% of Cu 2 O and 78.3% of CuI (Fig. 4h ). Electrochemical reduction of Cu_KX samples by LSV is expected to reduce all Cu(I) species to Cu 0 . The converted EDS data reveal (Fig. 4g, h ), however, that 0.33% of CuBr and 0.12% of CuI remains on the surface of the respective catalysts with the Cu_KI sample having a relatively higher content of Cu 2 O (22.7%) than either the Cu_KCl or Cu_KBr samples (<10%). More detailed analysis of residual halide using XPS and EDS are shown in Supplementary Figs. 12 and 13 . After electrochemical reduction, the high content of Cu 2 O in the Cu_KI is likely due to re-oxidation of the surface upon exposure to air during the time between sample preparation and EDS measurement (<30 min) and indicates that reduced Cu_KI is particularly susceptible to re-oxidation by air. This conclusion is consistent with the fact that Cu_KI undergoes abrupt morphological and chemical changes when electrochemically reduced by LSV, which generates a high density of under-coordinated atoms on the surface of the catalyst. Furthermore, this conclusion is supported by the work of Lum et al., where oxide-derived (OD) Cu with a high density of grain boundaries, could be re-oxidized very quickly when exposed to ambient air and moisture [34] . The chemical composition of electropolished Cu does not change significantly when immersed in air-saturated KHCO 3 for 10 min and subsequently electrochemically reduced by LSV as shown in the converted EDS data (Fig. 4e ). The percentage of Cu 2 O at electropolished Cu, however, does increase slightly from 1.7 to 2.9% upon immersion in air-saturated KHCO 3 for 10 min. This slight increase in Cu 2 O occurs via the oxidation reaction predicted by the Pourbaix diagram for copper [22] , [49] : 
    2 Cu ( s) + OH^ -  ( aq) ↔Cu_2O ( s) + 2e^ -  ( aq) + H^ +  ( aq)
 (5) As such, this reaction is likely to be a weak but important driving force that enables electrocatalysts to maintain a small amount of C + and subsurface oxygen despite the highly negative potentials used for electrochemical CO 2 RR. The mechanism by which Cu + species are stable to conditions used for CO 2 RR, however, remains indeterminate [12] . Nevertheless, because basic pH favors the oxidation reaction that forms Cu 2 O [Eq. ( 5 )] (i.e., hydroxide ions are consumed and protons are released), the rate of this reaction is enhanced during the electrochemical CO 2 RR, where protons are consumed and the pH near the electrode increases significantly. Thus, when a catalyst has defect sites that are susceptible to re-oxidation (e.g., oxide-derived Cu [11] or plasma-activated Cu [12] ), the oxidation reaction [Eq. ( 5 )] will generate C + and subsurface oxygen at those defect sites where the local pH is high during the electrochemical CO 2 RR. Notably, Lum et al. found that oxygen species of oxide-derived Cu are unstable and reduced at the highly negative potential, however, the rapid re-oxidation of Cu possessing a high density of defect sites occurs merely by soaking in 0.1 aqueous KHCO 3 electrolyte [34] . Their observation is consistent with Eq. ( 5 ) that basic pH of the electrolyte oxidizes Cu. Evaluating catalyst performance for electrochemical CO 2 RR To test the activity and selectivity of the halogenated Cu catalysts, bulk electrolysis of CO 2 was performed at a constant potential in CO 2 -saturated 0.1 M KHCO 3 for 40 min. Electrochemical CO 2 RR experiments were performed over a potential range from −1.1 to −2.1 V vs. Ag/AgCl (with iR -compensation these potentials correspond to −1.1 to −1.78 V vs. Ag/AgCl or −0.50 to −1.18 V vs. RHE). The resulting potential-dependent FEs from these experiments are shown in Fig. 5 . The catalysts were prepared via anodic halogenation of a Cu foil for different lengths of time (i.e., 100 s for Cu_KCl, 60 s for Cu_KBr, and 1 s for Cu_KI) to ensure complete coverage of the Cu substrate with Cu(I) halide (see Supplementary Figs. 4 – 6 ). 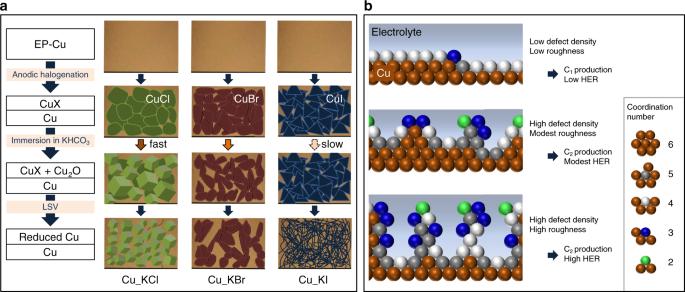Fig. 1: Schematics showing morphology of Cu catalysts. aThe method used to prepare Cu catalysts for electrochemical CO2RR: anodic halogenation in KX solutions where X = halogen, oxide formation in basic KHCO3, and electroreduction in neutral KHCO3by LSV. EP-Cu corresponds to electropolished Cu foils, LSV corresponds to linear sweep voltammetry.bTwo-dimensional visualization of under-coordinated Cu atoms and surface roughness with the corresponding outcomes when used for the electrochemical CO2RR. This schematic is simplified but face-centered cubic Cu has a coordination number of 12. The major product obtained on Cu(I)-halide-derived catalysts was C 2 H 4 , with its highest FE (45.1% on Cu_KCl, 49.5% on Cu_KBr, and 44.5% on Cu_KI) observed at ~ −1.15 V vs. RHE (see Table 1 ). For comparison, the major product obtained on electropolished Cu was CH 4 , with its highest FE (54.0%) at the same potential. Moreover, the Cu(I)-halide-derived catalysts produced CO with FEs in the range of 23–28% at potentials as low as ~ −0.68 V vs. RHE whereas electropolished Cu at this potential yielded CO with a FE of only 0.5%. Adsorbed CO (*CO) is an important intermediate required for production of C 2 and C 3 products via C–C bond coupling. The rate of reaction to produce C 2 H 4 is second order with respect to the surface concentration of adsorbed CO (*CO). Thus, a high density of active sites on the surface of the catalyst is necessary to produce a high surface concentration of *CO. Fig. 5: Performance of catalysts for electrochemical CO 2 reduction reaction. Potential-dependent faradaic efficiency of the products from the CO 2 RR products on electropolished Cu ( a ), chlorinated Cu ( b ), brominated Cu ( c ), and iodinated Cu ( d ). Anodic halogenation of Cu was performed in 0.1 M KCl at 1.1 V vs. Ag/AgCl for 100 s ( b ); in 0.1 M KBr at 0.18 V vs. Ag/AgCl for 60 s ( c ); in 0.1 M KI at −0.2 V vs. Ag/AgCl for 1 s ( d ). e – h FEs of C 1 , C 2 , and C 3 products from the same results shown in the corresponding upper plot. C 1 products include CO, formate, and CH 4 . C 2 products include C 2 H 4 , ethanol, acetate, acetaldehyde, and glycolaldehyde. C 3 products include n-propanol, propionaldehyde, and allyl alcohol. Data were acquired during 40 min of electrochemical CO 2 RR at a constant potential in 0.1 M KHCO 3 saturated with CO 2 . FE is shown as a function of the iR-corrected potential in RHE scale. Data legends apply to all plots in the same row. Source data are provided as a Source data file. Full size image Table 1 Representative FEs of products from electrochemical CO 2 RR shown in Figs. 5 and 6 . Full size table The effect of anodic halogenation time on CO 2 RR performance also was investigated (Fig. 6 ). All data shown in Fig. 6 were collected at −1.11 V vs. RHE, where the FE for H 2 was the lowest amongst all applied potentials studied. Supplementary Figs. 4 – 6 reveals that the underlying electropolished Cu substrate is exposed when anodic halogenation is performed for short periods of time. Thus, the Cu_KX catalysts produced by anodic halogenation for a short reaction time showed relatively high amounts of CH 4 and low amounts of C 2 H 4 and H 2 , a product distribution expected from electropolished Cu. Thus, to completely cover the underlying Cu substrate by Cu(I) halide, anodic halogenation needs to be applied for at least 60 s for Cu_KCl, 60 s for Cu_KBr and 5 s for Cu_KI. For these reaction times, 3.82, 0.80, and 0.028 C cm −2 of charge per unit area of electrode was used to make CuCl, CuBr, and CuI layers on electropolished Cu, respectively. The amount of charge vs. different amounts of time used for anodic halogenation is shown in Supplementary Fig. 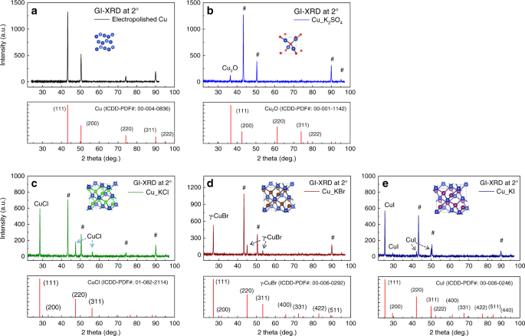Fig. 2: Crystal structures of halogenated Cu identified by grazing incident X-ray diffraction. GI-XRD patterns of the original electropolished Cu foil (a). Cu foils oxidized in 0.05 M K2SO4at 1.1 V vs. Ag/AgCl for 300 s (control sample) (b), or halogenated in KCl (c), in KBr (d), and in KI (e) for 100, 60, and 30 s, respectively. The symbol # indicates peaks corresponding to the underlying Cu-foil substrate. The incidence angle used for GI-XRD was 2°. The inset of each GI-XRD plot is a diagram of the unit cell for Cu, Cu2O, CuCl, CuBr, and CuI, from (a) to (e), respectively. Cu atoms are represented as blue spheres. Source data are provided as a Source data file. 14 . A relatively short amount of time of anodic halogenation covers the Cu substrate with CuI because iodide ions have a high ligand affinity for Cu [45] , [46] and the resulting CuI is highly stable [42] . In contrast, anodic chlorination or bromination of Cu requires more time to completely cover the Cu surface. Fig. 6: Effect of halogenation time on the performance of the catalysts for CO 2 reduction reaction. FEs of the products from electrochemical CO 2 RR are shown versus the amount of time the Cu foils were subjected to anodic halogenation in KCl ( a ), KBr ( b ), and KI ( c ). d – f FEs of H 2 , C 1 , C 2 , and C 3 products from the same results shown in the corresponding upper plot. 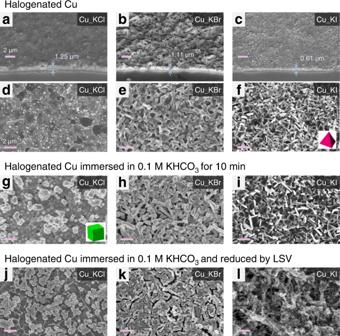Fig. 3: Morphology of halogenated Cu-foil electrodes. SEM images of halogenated Cu foils:a–fas-prepared;g–iafter immersion in 0.1 M KHCO3for 10 min;j–lafter reduction by LSV in the potential range from OCP to −1.8 V in CO2-saturated 0.1 M KHCO3.a–cCross-sectional images taken at a tilt angle of 45° to reveal the thickness of halogenated Cu.d–lPlan-view images. Anodic halogenation of Cu was performed for 50 s in 0.1 M KCl at 1.1 V (a,d,g,j); in 0.1 M KBr at 0.18 V (b,e,h,k); in 0.1 M KI at −0.2 V (c,f,i,l). All voltages are reported vs. Ag/AgCl. Scale bars: 2 μm. Data were acquired during 40 min of electrochemical CO 2 RR at a constant potential of ~ −1.11 V vs. RHE in 0.1 M KHCO 3 saturated with CO 2 . Data legends apply to all plots in the same row. 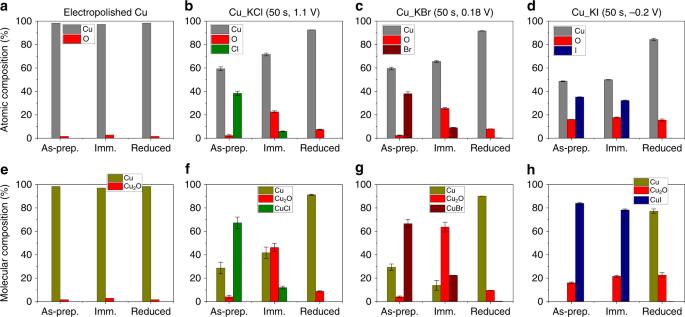Fig. 4: Energy-dispersive X-ray spectroscopy. a–dRaw data of atomic composition of electropolished Cu foil and halogenated Cu foils as measured by EDS.e–hCompositions of molecular species from converted EDS data. ‘As-prep.’ indicates the as-prepared catalyst by electropolishing or anodic halogenation. ‘Imm.’ indicates the catalyst underwent oxide formation by immersion in air-saturated 0.1 M KHCO3electrolyte for 10 min. ‘Reduced’ indicates the catalyst was reduced in CO2-saturated 0.1 M KHCO3electrolyte by LSV from its corresponding OCP to −1.8 V vs Ag/AgCl at a scan rate of 5 mV/s. Source data are provided as a Source data file. 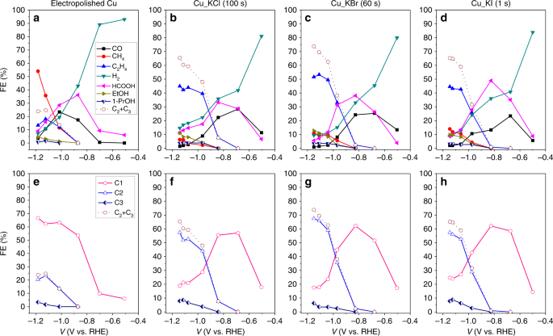Fig. 5: Performance of catalysts for electrochemical CO2reduction reaction. Potential-dependent faradaic efficiency of the products from the CO2RR products on electropolished Cu (a), chlorinated Cu (b), brominated Cu (c), and iodinated Cu (d). Anodic halogenation of Cu was performed in 0.1 M KCl at 1.1 V vs. Ag/AgCl for 100 s (b); in 0.1 M KBr at 0.18 V vs. Ag/AgCl for 60 s (c); in 0.1 M KI at −0.2 V vs. Ag/AgCl for 1 s (d).e–hFEs of C1, C2, and C3products from the same results shown in the corresponding upper plot. C1products include CO, formate, and CH4. C2products include C2H4, ethanol, acetate, acetaldehyde, and glycolaldehyde. C3products include n-propanol, propionaldehyde, and allyl alcohol. Data were acquired during 40 min of electrochemical CO2RR at a constant potential in 0.1 M KHCO3saturated with CO2. FE is shown as a function of the iR-corrected potential in RHE scale. Data legends apply to all plots in the same row. Source data are provided as a Source data file. Source data are provided as a Source data file. Full size image When the halogenation reaction time is increased up to 300 s, the FE for H 2 on all three Cu(I)-halide-derived catalysts increases significantly (i.e., FE for H 2 was 17.4% on Cu_KCl, 15.1% on Cu_KBr, and 19.9% on Cu_KI). To minimize the competing HER reaction, an optimal halogenation time was sought for each Cu_KX catalyst. The Cu_KCl catalyst that generated C 2 H 4 with a FE of 50.2% and C 2+ products with a FE of 70.7% was prepared using an anodic chlorination time of 60 s. Likewise, the Cu_KBr catalyst that generated C 2 H 4 with a FE of 50.9% and C 2+ products with a FE of 71.5% was prepared using an anodic bromination time of 90 s and the Cu_KI catalyst that generated C 2 H 4 with a 50.0% and C 2+ products with a FE of 72.6% was prepared using an anodic iodination time of only 10 s (see Table 1 ). Roughness factor, local pH, and competing HER Anodic halogenation generates a high density of active sites, which can be crystal grain boundaries or defect sites such as step atoms or under-coordinated atoms. 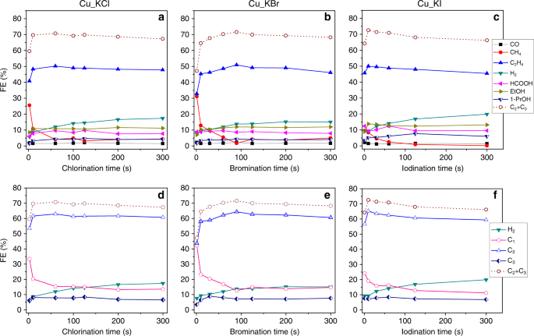Fig. 6: Effect of halogenation time on the performance of the catalysts for CO2reduction reaction. FEs of the products from electrochemical CO2RR are shown versus the amount of time the Cu foils were subjected to anodic halogenation in KCl (a), KBr (b), and KI (c).d–fFEs of H2, C1, C2, and C3products from the same results shown in the corresponding upper plot. Data were acquired during 40 min of electrochemical CO2RR at a constant potential of ~ −1.11 V vs. RHE in 0.1 M KHCO3saturated with CO2. Data legends apply to all plots in the same row. Source data are provided as a Source data file. These active sites in turn increase the production of C 2 products from CO 2 RR. If halogenation time is too long, however, the competing HER increases because the surface of the catalyst becomes too rough (see Supplementary Scheme 1 ). The roughness factor of an electrocatalyst can be determined by the double-layer (DL) capacitance method with the assumption that the surface charge is constant across different kinds of catalysts (see Supplementary Fig. 15 ). 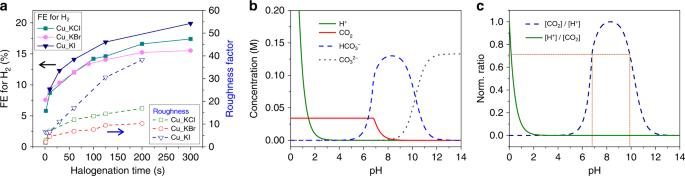Fig. 7: Relation between surface roughness of the electrocatalysts and HER. aThe roughness factor of the catalyst was estimated from the double-layer capacitance as measured by cyclic voltammetry (CV) in the potential range from −0.35 to −0.5 V vs. Ag/AgCl. FE for H2from Fig.6.bCalculated concentrations of reactants and buffering ions in 0.1 M KHCO3saturated with CO2.cThe normalized concentration ratio of dissolved CO2to proton as calculated from Fig.7b. Source data are provided as a Source data file. Figure 7a shows the relative roughness of Cu_KX as measured by DL capacitance, which are related as: 
    roughness factor = DL capacitance of the catalyst / 
    DL capacitance of the electropolished Cu
 Higher surface roughness promotes more HER. Figure 7a shows the relationship between the roughness of the catalysts, FE for H 2 , and halogenation time. This correlation between roughness and HER can be explained by a decrease in the concentration ratio of dissolved CO 2 to proton ([CO 2 ]/[H + ]) near the surface of the catalyst at high local pH. Although the buffering capacity of the bicarbonate electrolyte minimizes any increase in pH, the high current density observed at catalysts with high roughness rapidly depletes protons in the interfacial region and leads to a high local pH [17] , [22] . With high local pH, dissolved CO 2 becomes bicarbonate and carbonate ions by the equilibrium reaction shown in Eq. ( 2 ). The concentrations of dissolved CO 2 , bicarbonate and carbonate ions, and protons in the electrolyte were calculated and are shown in Fig. 7b (details on this calculation are given in Supplementary Information and shown in Supplementary Fig. 16 ). The normalized concentration ratio of [CO 2 ]/[H + ] (and its inverse) is shown in Fig. 7c , which at pH 6.8 and 9.9 is 0.706. In contrast, the maximum concentration ratio of [CO 2 ]/[H + ] occurs at pH 8.3. Above pH 9.9, the concentration ratio of [CO 2 ]/[H + ] decreases rapidly so that HER is favored over electrochemical CO 2 RR. In other words, a catalyst with higher roughness produces a higher current density in electrochemical CO 2 RR. A high current density rapidly consumes reactants, which are dissolved CO 2 and protons in the interfacial region between the catalyst and the electrolyte. The rapid consumption of protons results in a rise in the local pH. A high local pH decreases the concentration ratio of dissolved CO 2 to proton ([CO 2 ]/[H + ]) at the interfacial region by the equilibrium reaction [Eq. ( 2 )]. Consequently, a lower [CO 2 ]/[H + ] at a pH above 9.9 favors the competing HER side reaction. Data taken from the literature and included in Supplementary Fig. 17 also reveals a strong correlation between the roughness of the catalyst and the amount of HER. Our observation that mitigation of the rise of local pH suppresses HER is consistent with the previous report by Singh et al. [50] . Fig. 7: Relation between surface roughness of the electrocatalysts and HER. a The roughness factor of the catalyst was estimated from the double-layer capacitance as measured by cyclic voltammetry (CV) in the potential range from −0.35 to −0.5 V vs. Ag/AgCl. FE for H 2 from Fig. 6 . b Calculated concentrations of reactants and buffering ions in 0.1 M KHCO 3 saturated with CO 2 . c The normalized concentration ratio of dissolved CO 2 to proton as calculated from Fig. 7b . Source data are provided as a Source data file. Full size image Hori et al. studied single-crystal Cu with a (911) facet introduced a (111) step for every five (100) basal planes [5(100) × (111)] [20] . The performance of this facet in the electrochemical CO 2 RR was superb, producing H 2 at a FE of 12.7%, C 2 H 4 at a FE of 50.9% and C 2+ products at a FE of 79.5% at a stir rate of 260 rpm [in comparison to polycrystalline Cu, which in our hands produces H 2 at a FE of 15.1%, C 2 H 4 at a FE of 20.4% and C 2+ products at a FE of 32.6% with a comparable rate of stirring (~290 rpm)]. However, producing single-crystal catalysts at a scale required for carbon utilization is not economically or technically feasible. Thus, a simple and inexpensive alternative to single-crystal Cu is to prepare Cu catalysts via anodic halogenation. More recent studies have proposed the predominant facet (100) of cubic structures of Cu promotes the conversion of CO 2 into multi-carbon products [14] , [19] . Although Cu_KCl exhibits cubic structures on its surface, both Cu_KBr and Cu_KI have irregular microstructures (see Fig. 3 ). All three Cu_KX catalysts, however, have a high density of defect sites and produce C 2+ products with FEs up to 70.73% on Cu_KCl, 71.54% on Cu_KBr, and 72.58% on Cu_KI. Thus, in addition to specific crystal facets, a high density of defect sites (i.e., step sites and low-coordinated Cu atoms) is essential for converting CO 2 into C 2 products via electrochemical CO 2 RR at a Cu catalyst. This finding is consistent with the results of Hori et al. that Cu (100) single crystal is not an ideal facet for selective C 2+ production (FE CH4 = 30.4% and FE C2H4 = 40.4%) [20] and the more recent claim that the presence of oxygen species in surface and subsurface regions of catalysts with nano-cubic morphology are more important for achieving high activity and selectivity for C 2+ hydrocarbons or alcohols than the presence of Cu(100) facets themselves [13] . Anodic halogenation of electropolished Cu followed by surface reconstruction from base-induced oxide formation and electroreduction creates a surface with a high density of defect sites. These sites stabilize species such as Cu + and subsurface oxygen, which are known to promote C 2+ production during the electrochemical CO 2 RR. Evidence of a high density of defect sites on the surface of Cu_KX catalysts is provided by incidence-angle dependent GI-XRD data (Supplementary Fig. 18 ), which shows decreased crystal ordering at the surface of Cu_KBr during surface reconstruction. Furthermore, EDS data reveals the high susceptibility of these surfaces to re-oxidation. The density of defect sites in oxide-derived Cu has recently been determined using positron annihilation spectroscopy (PAS) [35] . Based on our results, we conclude that a high density of defect sites is the most important attribute of a Cu catalyst that selectively converts CO 2 into C 2+ products via the electrochemical CO 2 RR. Interestingly, ethane (C 2 H 6 ) is produced when the roughness factor exceeds 30 (FE C2H6 = ~1.2% in this work). The mechanistic pathway to produce C 2 H 6 has been proposed to be the reaction between adsorbed ethylene (*C 2 H 4 ) and adsorbed hydrogen (*H) [51] . Therefore, observation of C 2 H 6 indicates high surface concentrations of both *C 2 H 4 and *H, which only can be attributed to a high density of defect sites and high roughness, respectively. Thus, production of C 2 H 6 indicates that the roughness of the catalyst needs to be lowered to obtain the optimal balance of a high density of defect sites that favors C 2 H 4 production and low roughness that suppresses HER. Recently, Wang et al. reported a wet-chemistry method to prepare cuprous-halide-derived catalysts with FE up to 58% for C 2+ product [52] . Our study significantly advances this reaction to obtain a FE of 72.6% for C 2+ product. This advance is made possible by the discovery that features of Cu catalysts can be optimized for this reaction (e.g., defect density, roughness) by controlling the duration of anodic halogenation at a constant potential. Our study also highlights the importance of the correlation between the roughness of the catalyst and HER and the impact of that correlation on electrochemical CO 2 RR at negative potentials (~ −1 V vs. RHE). Thus, the [CO 2 ]/[H + ] ratio provides an important parameter that can be controlled to yield a catalyst that is both efficient and selective for C 2+ products. In summary, Cu(I)-halide-derived catalysts were prepared using anodic halogenation. The optimal time and voltage for anodic halogenation was 60–100 s at 1.1 V, 60–90 s at 0.18 V, and 10 s at −0.2 V vs. Ag/AgCl for Cu_KCl, Cu_KBr, and Cu_KI, respectively. Iodide ions react with the Cu surface rapidly at weak oxidative potentials because of the high affinity of I − to form CuI. All Cu(I)X-derived catalysts (where X = Cl, Br, or I) were found to be excellent catalysts for producing C 2+ products via the electrochemical CO 2 RR with FE C2+ of 70.7%, 71.5%, and 72.6% on Cu_KCl, Cu_KBr, and Cu_KI, respectively. By exploiting volume changes that occur during anodic halogenation and subsequent surface reconstruction, we show that anodic halogenation is a simple to perform and scalable method for consistently preparing Cu catalysts with a high density of surface defect sites and low roughness. The high density of defect sites promotes production of multi-carbon products and the low roughness suppresses the competing HER. These results, taken together, provide an approach to preparing catalysts for efficient conversion of CO 2 to C 2+ products that has characteristics desirable for carbon utilization technologies: simple to perform, consistent, regenerative, and scalable. Preparation of electrocatalysts All Cu foils were mechanically polished with 400 grit sandpaper, and rinsed with deionized (DI) water. The Cu foils (2 × 5 cm 2 ) subsequently were electropolished by chronoamperometry in 85% phosphoric acid at 1.5 V with a Cu counter electrode in a two-electrode configuration. The electropolished Cu foils were rinsed with DI water. After cutting the electropolished Cu foils into 2 × 0.5 cm 2 pieces, the foils were flattened and both the back side and part of the front side were covered with polyimide (PI) tape to define the geometric area of the working electrode. The electrode was wrapped in PTFE tape (Swagelok) to prevent detachment of the PI tape. The exposed geometric area was typically 0.35 cm 2 . KCl (Macron fine chemicals), KBr (Fisher Scientific), and KI (Fisher Scientific) were dissolved in DI water to a concentration of 0.1 M. Anodic chlorination, bromination, and iodination was performed on an electropolished Cu foil immersed in 0.1 M KCl, KBr, and KI at 1.1, 0.18, and −0.2 V vs. Ag/AgCl, respectively, in a three-electrode configuration using a potentiostat (Pine Instrument Company, Biopotentiostat, model AFCBP1). The counter electrode was Pt gauze and the reference electrode was Ag/AgCl (saturated KCl) electrode. The OCP of electropolished Cu in 0.1 M KCl, KBr, and KI was −0.115, −0.134, and −0.315 V vs. Ag/AgCl, respectively (Supplementary Fig. S1 ). Characterization of the electrocatalysts SEM images were acquired using a LEO 1530 VP ultra-high resolution field emitter SEM at 10 kV. Elemental analysis of samples was obtained using the EDS accessory (Oxford Instruments, Inca X-sight, model 7426) of the SEM. The GI-XRD data were obtained using a Bruker D8 Discovery High resolution X-ray Diffractometer at incidence angle of 2° and wavelength of 1.54 Å. The double-layer capacitance was measured by cyclic voltammetry in the potential range from −0.35 to −0.5 V vs. Ag/AgCl in CO 2 -saturated 0.1 M KHCO 3 after electrochemical CO 2 RR. XPS equipment of PHI 5000 VersaProbe (Ulvac-PHI, Japan) was used to characterize the surface of the Cu catalysts. Electrochemical CO 2 reduction Electrochemical CO 2 RR was carried out in a custom made two compartment cell, separated by a Nafion 117 proton-exchange membrane. The two compartments were filled with 8.2 ml of 0.1 M KHCO 3 (Sigma-Aldrich, ≥99.95%) electrolyte. A three-electrode configuration was employed: Cu-foil working electrode, Pt gauze counter electrode, and a home-built Ag/AgCl reference electrode. The working and reference electrodes were placed in the cathode compartment and the Pt gauze counter electrode was placed in the anode compartment. Prior to initiating electrochemical CO 2 RR, the halogenated Cu-foil electrode was immersed in 0.1 M KHCO 3 electrolyte and linear sweep voltammetry was performed with a scan rate of 5 mV/s from the OCP to the working potential (usually −0.2 to −2.1 V vs Ag/AgCl). Subsequently, CO 2 RR was performed with fresh electrolyte saturated with CO 2 . Before and during electrochemical CO 2 RR, the cell was purged continuously with CO 2 at a flow rate of 20 mL/min as measured with a rotameter (OMEGA FL-3841G FT-032-41-GL-VN). Electrochemical CO 2 RR was performed by chronoamperometry for 40 min with a magnetic stirring bar spinning at ~1500 rpm. A Thermolyne Nuova stir plate (model No. SP18425) was used to stir a 1-cm-long magnetic bar in the electrolyte. The stirring speed was calibrated in comparison with the Fisher Scientific hot plate/stirrer (Cat. No. 11-100-49SH). It is worth noting that all experimental results on electrochemical CO 2 RR were obtained while stirring the electrolyte with a magnetic stirrer at ~1500 rpm. After electrochemical CO 2 RR, the solution resistance ( R ) was measured with a potentiostatic electrochemical impedance spectrometer (Solartron, 1255 HF Frequency Response Analyzer) at 10 kHz. All electrochemical data was collected vs. Ag/AgCl reference. The iR -compensated potentials relative to the reversible hydrogen electrode (RHE) are shown in the tables in the supporting information using the following equations: 
    V_comp( Ag/AgCl)=V_appl( Ag/AgCl)+iR
 
    V_comp( RHE)=V_comp( Ag/AgCl)+0.197+0.059 ∗pH
 Liquid-phase products in the catholyte were collected for quantification using nuclear magnetic resonance (NMR). Product analysis The reduction compartment of the gas-tight reactor was connected to the inlet of the sample loop of a gas chromatograph (GC, Buck Scientific, Model 910). GC measurements were performed on sample injections taken after 10 and 38 min of the CO 2 RR to determine the concentration of gaseous products present: CO, CH 4 , C 2 H 4 , H 2 . The GC was equipped with a methanizer and a flame ionization detector (FID) to detect CO and hydrocarbons and a thermal conductivity detector (TCD) to detect H 2 . Nitrogen was used as the carrier gas. Liquid products were quantified using 1D 1 H NMR (400 MHz, Bruker high field NMR spectrometers). Each sample of catholyte (700 μL) was mixed with 35 μL of a D 2 O solution containing internal standards: 50 mM phenol and 10 mM dimethyl sulfoxide (DMSO). The water peak was suppressed by a WET procedure (Bruker). The acquired NMR data were processed with Topspin 4.0.5 software. The peak area of the liquid product (formate) at higher chemical shift with respect to the suppressed water peak (chemical shift = 4.7 ppm) was normalized to the peak area of phenol (chemical shift = 7.2 ppm). The peak areas of the liquid products (acetate, ethanol, propanol, acetaldehyde, propionaldehyde, glycolaldehyde, and allyl alcohol) at lower chemical shift with respect to the suppressed water peak were normalized to the peak area of DMSO (chemical shift = 2.6 ppm).